Apical membrane antigen 1 mediates apicomplexan parasite attachment but is dispensable for host cell invasion Apicomplexan parasites invade host cells by forming a ring-like junction with the cell surface and actively sliding through the junction inside an intracellular vacuole. Apical membrane antigen 1 is conserved in apicomplexans and a long-standing malaria vaccine candidate. It is considered to have multiple important roles during host cell penetration, primarily in structuring the junction by interacting with the rhoptry neck 2 protein and transducing the force generated by the parasite motor during internalization. Here, we generate Plasmodium sporozoites and merozoites and Toxoplasma tachyzoites lacking apical membrane antigen 1, and find that the latter two are impaired in host cell attachment but the three display normal host cell penetration through the junction. Therefore, apical membrane antigen 1, rather than an essential invasin, is a dispensable adhesin of apicomplexan zoites. These genetic data have implications on the use of apical membrane antigen 1 or the apical membrane antigen 1–rhoptry neck 2 interaction as targets of intervention strategies against malaria or other diseases caused by apicomplexans. Most apicomplexans, including the agents of malaria ( Plasmodium ) and toxoplasmosis ( Toxoplasma ), are obligate intracellular parasites. Many invade host cells by a conserved mechanism involving the formation of a zone of tight attachment between the parasite apex and the host cell [1] , called tight junction (TJ). The current view is that the TJ is primarily a molecular bridge between the parasite sub-membrane actin-myosin motor and a stable and stationary [2] anchor associated with the host cell surface/cortex, which allows parasite traction into a parasitophorous vacuole (PV) within the host cell [3] , [4] . The transmembrane protein apical membrane antigen 1 (AMA1), arguably the most studied protein in the Apicomplexa phylum and a long-standing malaria vaccine candidate, is thought to shape the TJ on the parasite side [5] , [6] , [7] , [8] , [9] , [10] , [11] . The cytoplasmic tail of AMA1 was reported to bind aldolase [8] in vitro , considered a signature of proteins that bind parasite actin and the motor [12] , [13] . The ectodomain of AMA1 tightly binds in parasite extracts to the rhoptry neck 2 (RON2) protein [9] , [10] , a protein secreted from the parasite rhoptries that specifically localizes at the TJ, where it inserts in the host cell membrane and is presumably linked to the cell cortical cytoskeleton via other RON proteins, like RON4. Moreover, antibodies or peptides that inhibit the AMA1–RON2 interaction drastically reduce host cell invasion by Plasmodium merozoites [14] , [15] , [16] and Toxoplasma tachyzoites [9] , [10] . T. gondii or P. falciparum AMA1 bound to RON2 peptide were co-crystalized, revealing a conserved RON2 loop inserting deep into an AMA1 hydrophobic groove [17] , [18] . This reinforced the model of this interaction constituting the traction point used by the parasite to power the active internalization inside the PV [19] , [20] , [21] , and led to the proposal of developing broad-spectrum small-molecule inhibitors of apicomplexan invasion targeting the AMA1–RON2 interaction [22] , [23] , [24] . In addition, AMA1 has been reported to be involved in rhoptry secretion [15] , [25] as well as for providing a signal initiating intracellular replication [26] . Recently, P. berghei and T. gondii parasites in which AMA1 was silenced ( AMA1 knockdown, AMA1 KD ) were found to remain competent for shaping a TJ and invading host cells [27] . However, as AMA1 KD parasites might still express residual levels of AMA1, these data were not considered as challenging any of the proposed roles of AMA1 in invasion [18] , [23] , [28] , [29] . In agreement with an essential role of AMA1 at some stage of the parasite invasion process, all attempts to inactivate AMA1 in both Plasmodium [30] , [31] and Toxoplasma [32] have failed so far. Here, we report the inactivation of AMA1 in the tachyzoite of T. gondii , which invades virtually any cell type in the host, and in the merozoite and sporozoite stages of P. berghei , which invade erythrocytes and hepatocytes, respectively. AMA1 was deleted from the parasite genome by the diCre- loxP recombination approach in T. gondii and by direct homologous recombination in P. berghei . All three AMA1 knockout (AMA1 KO ) zoites are still capable of penetrating the respective host cell like the wild type (WT). Tachyzoites and merozoites, however, display a defect in host cell binding. These genetic data indicate that AMA1 and the RON proteins act separately during apicomplexan invasion, and that the AMA1–RON2 interaction does not have an essential role at the TJ. Role of AMA1 in T. gondii tachyzoite infection of host cells To investigate the role of AMA1 in T. gondii tachyzoites, we generated AMA1 KO parasites using the diCre- loxP site-specific recombination system [33] . The loxP AMA1 loxP -YFP-HXGPRT construct ( Fig. 1a ) was inserted in the ku80::diCre strain, which encodes two inactive fragments of Cre fused to rapamycin-binding proteins. Upon rapamycin addition and Cre reconstitution, recombinant parasites excise AMA1 ( Fig. 1b ) and express YFP . An excised clone, called TgAMA1 KO , which does not produce AMA1 as shown by western blot ( Fig. 1c ) and immunofluorescence ( Fig. 2a ) analysis, was selected and maintained using routine culture procedures. When measuring parasite infectivity by plaque assay, the plaque size is ~2 to 2.5 times smaller with TgAMA1 KO than control parasites ( Fig. 2a,b ), a rather mild phenotype. Reintroduction of internally tagged AMA1 FLAG in TgAMA1 KO parasites fully restores overall growth, demonstrating the specificity of the observed phenotype ( Fig. 2a ). Importantly, no significant difference can be noticed in the replicative rates ( Fig. 2c,d ), egress efficiency ( Fig. 2e ) or motility patterns ( Fig. 2f ) between TgAMA1 KO and control tachyzoites. Therefore, AMA1 is not involved in tachyzoite gliding, intravacuolar replication or egress from host cells. 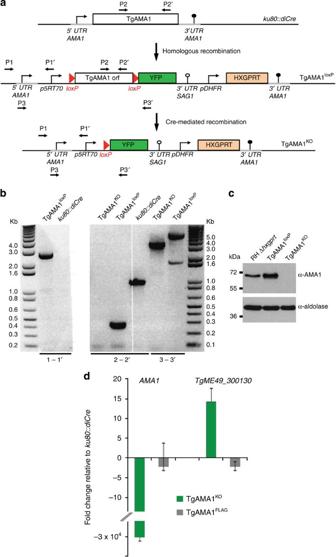Figure 1: Isolation of AMA1KOT. gondiitachyzoites using the diCre system. (a) Schematic illustration of the knockout strategy. Homology regions for recombination are depicted in grey flanking theloxPAMA1loxP-YFP-HXGPRT construct (second line). The endogenousAMA1in theku80::diCrestrain was replaced by a floxed (red arrows) copy of theAMA1open reading frame (ORF) followed byYFP-coding sequence to generate the TgAMA1loxPstrain. Cre-mediated recombination induced with rapamycin excised theAMA1ORF and activatedYFPexpression (TgAMA1KO). (b) Diagnostic PCR shows replacement of endogenousAMA1in TgAMA1loxPand excision ofAMA1upon Cre-mediated recombination. Primers are as illustrated ina. (c) Immunoblot analysis shows the absence of AMA1 (63 kDa) expression in TgAMA1KOparasites compared with RH Δhxgprtand TgAMA1loxPstrains. Anti-aldolase antibody was used for loading control. (d) Transcript levels ofAMA1and theAMA1homologueTgME49_300130in the clones TgAMA1FLAGor TgAMA1KOpropagated in continuous culture. Data are representative of four independent experiments from two RNA preparations and are shown as mean fold change±s.d. relative to transcript levels measured in theku80::diCrestrain. Figure 1: Isolation of AMA1 KO T. gondii tachyzoites using the diCre system. ( a ) Schematic illustration of the knockout strategy. Homology regions for recombination are depicted in grey flanking the loxP AMA1 loxP -YFP-HXGPRT construct (second line). The endogenous AMA1 in the ku80::diCre strain was replaced by a floxed (red arrows) copy of the AMA1 open reading frame (ORF) followed by YFP -coding sequence to generate the TgAMA1 loxP strain. Cre-mediated recombination induced with rapamycin excised the AMA1 ORF and activated YFP expression (TgAMA1 KO ). ( b ) Diagnostic PCR shows replacement of endogenous AMA1 in TgAMA1 loxP and excision of AMA1 upon Cre-mediated recombination. Primers are as illustrated in a . ( c ) Immunoblot analysis shows the absence of AMA1 (63 kDa) expression in TgAMA1 KO parasites compared with RH Δ hxgprt and TgAMA1 loxP strains. Anti-aldolase antibody was used for loading control. ( d ) Transcript levels of AMA1 and the AMA1 homologue TgME49_300130 in the clones TgAMA1 FLAG or TgAMA1 KO propagated in continuous culture. Data are representative of four independent experiments from two RNA preparations and are shown as mean fold change±s.d. relative to transcript levels measured in the ku80::diCre strain. 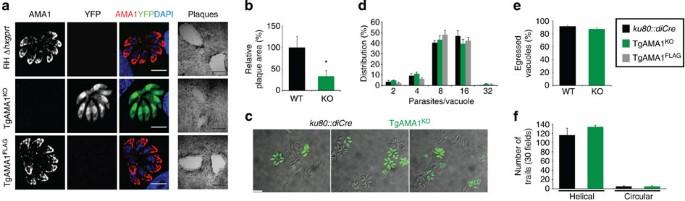Figure 2: Infection of cell monolayers by TgAMA1KOtachyzoites. (a) AMA1 immunostaining in RH Δhxgprt, TgAMA1KOor TgAMA1FLAGmultiplying inside host cells. Scale bar, 5 μm. Plaque assay with HFF cells after 6 days is shown on the right for each strain. Cells are stained with Giemsa. Scale bar, 0.5 mm. (b) Plaque area induced on HFF cells after 7 days infection with WT or TgAMA1KOtachyzoites. Mean area of ten plaques±s.d. is depicted, *P-value <0.0001 in unpaired Student’st-test. (c) Pictures of HFF cell monolayers 20 h after co-infection with theku80::diCre(non-fluorescent) and TgAMA1KO(green) strains. Scale bar, 10 μm. (d) Quantification of parasites per vacuole after cell infection. (e) Quantification of egressed vacuoles. Data show mean±s.d. of three independent experiments. (f) Analysis of motility patterns. Data represent the mean±s.d. of helical or circular trails associated with parasites counted in 30 fields of view. (b,d–f) The colour codes are shown in panele. DAPI, 4′,6-diamidino-2-phenylindole; KO, knockout. Full size image Figure 2: Infection of cell monolayers by TgAMA1 KO tachyzoites. ( a ) AMA1 immunostaining in RH Δ hxgprt , TgAMA1 KO or TgAMA1 FLAG multiplying inside host cells. Scale bar, 5 μm. Plaque assay with HFF cells after 6 days is shown on the right for each strain. Cells are stained with Giemsa. Scale bar, 0.5 mm. ( b ) Plaque area induced on HFF cells after 7 days infection with WT or TgAMA1 KO tachyzoites. Mean area of ten plaques±s.d. is depicted, * P -value <0.0001 in unpaired Student’s t -test. ( c ) Pictures of HFF cell monolayers 20 h after co-infection with the ku80::diCre (non-fluorescent) and TgAMA1 KO (green) strains. Scale bar, 10 μm. ( d ) Quantification of parasites per vacuole after cell infection. ( e ) Quantification of egressed vacuoles. Data show mean±s.d. of three independent experiments. ( f ) Analysis of motility patterns. Data represent the mean±s.d. of helical or circular trails associated with parasites counted in 30 fields of view. ( b , d – f ) The colour codes are shown in panel e . DAPI, 4′,6-diamidino-2-phenylindole; KO, knockout. Full size image We then investigated AMA1 KO tachyzoite invasion of host cells in more detail. When measured by fluorescence microscopy, TgAMA1 KO tachyzoite invasion efficiency is 30–40% that of the parental ku80::diCre strain ( Fig. 3a ). To investigate whether the pattern of TgAMA1 KO tachyzoite invasion of host cells is normal or altered, TgAMA1 KO tachyzoites invading human foreskin fibroblasts (HFFs) or normal rat kidney (NRK) fibroblasts were captured by confocal microscopy and analysed after three-dimensional reconstruction ( Fig. 3b ). Entering mutant zoites ( n =53) constantly display a typical RON4 circular staining around the parasite constriction site after cell permeabilization, indicating normal rhoptry secretion and TJ formation during invasion. In line with the normal gliding capacity of TgAMA1 KO tachyzoites, micronemal protein 2 (MIC2) [34] , which is secreted like AMA1 from the microneme organelles, is normally exposed on the surface of invading TgAMA1 KO tachyzoites ( Fig. 3b ). Moreover, video microscopy of invading TgAMA1 KO zoites shows that successful invasion follows a one go and smooth process with similar kinetics as controls ( Fig. 3c,d and Supplementary Movies 1–3 ), and in all cases ( n =20) a clear constriction site, suggestive of normal TJ, is observed. We conclude that in the tachyzoite AMA1 is not necessary for structuring a fully functional TJ, in which the RON proteins act independently of AMA1. 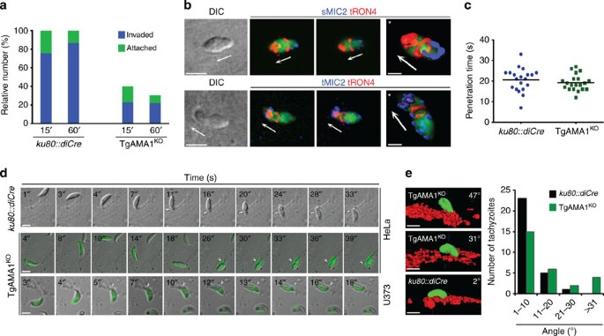Figure 3: Host cell invasion by TgAMA1KOtachyzoites. (a) Red/green invasion assay. Attached and invaded parasites were numerated and normalized to total number ofku80::diCre. Data show mean of a representative assay out of three independent experiments. At least 400 tachyzoites were counted for each strain. (b) Invading parasites stained with antibodies against the surface (sMIC2) or total (tMIC2) micronemal protein MIC2, and with anti-RON4 antibodies to mark the TJ. Scale bars, 5 μm. The right panels (*) show processed three-dimensional (3D) images. Scale bars, 2 μm. Arrows indicate the direction of movement. (c) Penetration kinetics. Twenty independent events for each strain were recorded by time-lapse microscopy. (d) Time lapses ofku80::diCre(upper row) or TgAMA1KO(green, bottom rows) tachyzoites invading epithelial cells (cell types are indicated on the right). Numbers indicate seconds and the white arrows show the constriction sites, characteristic of TJ formation. Scale bars, 5 μm. (e) 3D reconstruction of the positioning ofku80::diCreor AMA1KOtachyzoites with labelled SAG-1 (green) attached to host cells expressing a fluorescent marker at the plasma membrane (red). Scale bars, 5 μm. The plot shows the angle of the parasite in relation to the mCherry-expressing host cell membrane measured for 50 tachyzoites of each strain. DIC, differential interference contrast. Figure 3: Host cell invasion by TgAMA1 KO tachyzoites. ( a ) Red/green invasion assay. Attached and invaded parasites were numerated and normalized to total number of ku80::diCre . Data show mean of a representative assay out of three independent experiments. At least 400 tachyzoites were counted for each strain. ( b ) Invading parasites stained with antibodies against the surface (sMIC2) or total (tMIC2) micronemal protein MIC2, and with anti-RON4 antibodies to mark the TJ. Scale bars, 5 μm. The right panels (*) show processed three-dimensional (3D) images. Scale bars, 2 μm. Arrows indicate the direction of movement. ( c ) Penetration kinetics. Twenty independent events for each strain were recorded by time-lapse microscopy. ( d ) Time lapses of ku80::diCre (upper row) or TgAMA1 KO (green, bottom rows) tachyzoites invading epithelial cells (cell types are indicated on the right). Numbers indicate seconds and the white arrows show the constriction sites, characteristic of TJ formation. Scale bars, 5 μm. ( e ) 3D reconstruction of the positioning of ku80::diCre or AMA1 KO tachyzoites with labelled SAG-1 (green) attached to host cells expressing a fluorescent marker at the plasma membrane (red). Scale bars, 5 μm. The plot shows the angle of the parasite in relation to the mCherry-expressing host cell membrane measured for 50 tachyzoites of each strain. DIC, differential interference contrast. Full size image Next, we assessed tachyzoite adhesion to host cells. After 15 or 60 min incubation with live HFF cell monolayers, approximately two- to threefold fewer mutant versus control tachyzoites associate with host cells (total: extracellular attached and internalized combined), whereas three- to fourfold fewer mutants are located inside host cells, suggesting a primary defect of mutant zoites in host cell attachment ( Fig. 3a ). Importantly, about a third of the TgAMA1 KO tachyzoite population adopts a distinct position relative to the host cell than controls, by binding only via the apical end rather than throughout their length ( Fig. 3e ), like previously observed for AMA1 KD tachyzoites [27] . This confirms that AMA1 has an important role in tachyzoite adhesion to/positioning onto host cells before TJ formation, an event that favours, but is not required for, host cell invasion. Role of AMA1 in P. berghei merozoite infection of erythrocytes To inactivate AMA1 in P. berghei , WT ANKA blood stages were transfected with a construct designed to replace endogenous AMA1 by pyrimethamine-resistance and green-fluorescence cassettes ( Fig. 4a ). Dedicated in vivo selection protocols with several days of drug pressure reproducibly generated mixtures of targeted green fluorescent protein (GFP + ) AMA1 − parasites, that is, AMA1 KO , and non-targeted GFP − AMA1 + parasites, presumably spontaneous pyrimethamine-resistant mutants that typically emerge after long selection times. Southern blot analysis indicates the presence in the selected population of both the WT AMA1 locus and the expected allelic replacement ( Fig. 4b ). In agreement with this, immunofluorescence assays reveal erythrocytes infected by either GFP + AMA1 − or GFP − AMA1 + parasites ( Fig. 4c ). The multiplication rate of AMA1 KO parasites, assessed by co-injection with control red fluorescent protein (RFP + ) parasites [35] in mice and monitoring parasite multiplication by fluorescence-activated cell sorting (FACS), is ~35% that of RFP + parasites ( Fig. 4d ). As internalized AMA1 KO parasites generate normal numbers of progeny merozoites after a normal developmental cycle ( Fig. 4e ), that is, AMA1 is not important for merozoite replication inside erythrocytes, the decreased multiplication rate of AMA1 KO parasites reflects a defect in merozoite entry into erythrocytes. 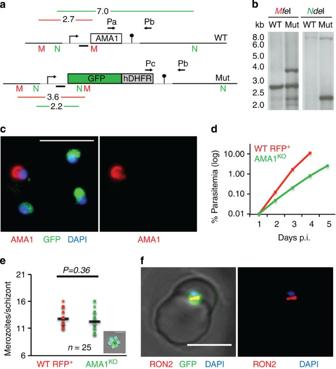Figure 4: Selectionin vivoofP. bergheiAMA1KOmerozoites. (a) Schematic illustration of the knockout strategy. Grey lines represent regions of homology for recombination. Integration of the targeting sequence disrupts theAMA1-coding sequence and replaces it by fluorescent (GFP) and drug resistance (hDHFR) markers. Pa, Pb and Pc: primers used for diagnostic PCR inFig. 8d. M,MfeI and N,NdeI: enzymes used for digestion before Southern blotting. Southern blotting probe is represented as a black line. (b) Southern blot analysis of theAMA1locus in wild-type (WT) ANKA strain and mutant (Mut) parasites. Digestion with the enzymesMfeI orNdeI produces fragments of different sizes for WT or mutant loci. (c) AMA1 immunostaining of GFP+(AMA1KO) and GFP−(pyrimethamine-resistant WT) merozoites. Scale bar, 10 μm. (d) Kinetics ofin vivogrowth of GFP+(AMA1KO) and WT RFP+(WT RFP) in co-infected mice. Parasitemia was assessed daily by FACS and plotted as the mean parasitemia measured in five mice. Data are representative of two independent experiments. (e) Number of merozoites per schizont formed 16 h afterin vitroincubation of erythrocytes infected with GFP+(AMA1KO) or WT RFP+ring stages. Only cells infected with a single parasite were counted. A picture of a cell infected with a GFP+(AMA1KO) schizont is shown in the plot. Scale bar, 5 μm.P=0.36 in one-way analysis of variance followed by Tukey HSD test. (f) RON2 immunostaining of a GFP+(AMA1KO) merozoite invading a host cell shows the formation of a RON2 ring, suggestive of a formed TJ. Scale bar, 5 μm. DAPI, 4′,6-diamidino-2-phenylindole. Figure 4: Selection in vivo of P. berghei AMA1 KO merozoites. ( a ) Schematic illustration of the knockout strategy. Grey lines represent regions of homology for recombination. Integration of the targeting sequence disrupts the AMA1 -coding sequence and replaces it by fluorescent ( GFP ) and drug resistance ( hDHFR ) markers. Pa, Pb and Pc: primers used for diagnostic PCR in Fig. 8d . M, Mfe I and N, Nde I: enzymes used for digestion before Southern blotting. Southern blotting probe is represented as a black line. ( b ) Southern blot analysis of the AMA1 locus in wild-type (WT) ANKA strain and mutant (Mut) parasites. Digestion with the enzymes Mfe I or Nde I produces fragments of different sizes for WT or mutant loci. ( c ) AMA1 immunostaining of GFP + (AMA1 KO ) and GFP − (pyrimethamine-resistant WT) merozoites. Scale bar, 10 μm. ( d ) Kinetics of in vivo growth of GFP + (AMA1 KO ) and WT RFP + (WT RFP) in co-infected mice. Parasitemia was assessed daily by FACS and plotted as the mean parasitemia measured in five mice. Data are representative of two independent experiments. ( e ) Number of merozoites per schizont formed 16 h after in vitro incubation of erythrocytes infected with GFP + (AMA1 KO ) or WT RFP + ring stages. Only cells infected with a single parasite were counted. A picture of a cell infected with a GFP + (AMA1 KO ) schizont is shown in the plot. Scale bar, 5 μm. P =0.36 in one-way analysis of variance followed by Tukey HSD test. ( f ) RON2 immunostaining of a GFP + (AMA1 KO ) merozoite invading a host cell shows the formation of a RON2 ring, suggestive of a formed TJ. Scale bar, 5 μm. DAPI, 4′,6-diamidino-2-phenylindole. Full size image We next characterized interactions between AMA1 KO merozoites and erythrocytes using imaging flow cytometry (IFC), which combines microscopy and flow cytometry and provides quantitative and functional information using imaging algorithms. Briefly (see Methods), after mixing mouse erythrocytes pre-stained with the lipid dye PKH26 with P. berghei GFP + merozoites [36] collected from synchronized schizont cultures, parasites interacting with a host cell are identified as GFP signals in a gated PKH26 + population ( Fig. 5a , left panel), and internalized parasites are further recognized by co-localization of GFP with an increased PKH26 signal relative to the rest of the cell ( Fig. 5b ), a labelling suggestive of merozoites surrounded by a tight-fitting vacuole membrane [37] ( Fig. 5a , right panel). Using control GFP + merozoites incubated for 10 min with PKH26-stained erythrocytes before fixation, ~43.8% score as ‘associated’ with erythrocytes (Ery A ; Fig. 5a , left panel), whereas ~3.8% score as ‘internalized’ inside erythrocytes (Ery I ; Fig. 5a , right panel). Importantly, cytochalasin D, which prevents merozoite internalization but not attachment to erythrocytes [38] , does not significantly affect the Ery A but drastically reduces the Ery I population ( Fig. 5a,c ), which validates the Ery I population algorithm. Using merozoites of the AMA1 KO -containing population, ~8.6% of the GFP + AMA1 KO merozoites score as Ery A and ~0.48% as Ery I ( Fig. 5d ). A similar reduction relative to control merozoites is obtained when samples are fixed after 3 min incubation ( Fig. 5e ), indicating a primary defect in adhesion of AMA1 KO merozoites. Like AMA1 KO tachyzoites, AMA1 KO merozoites form a normal RON (RON2) ring during host cell invasion ( Fig. 4f ). 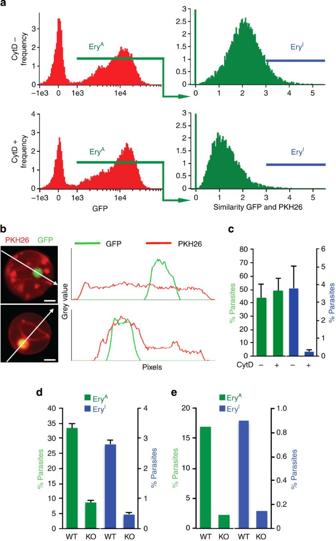Figure 5: IFC analysis of erythrocyte invasion by AMA1KOmerozoites. (a) WT GFP+merozoites isolated from blood cultures were incubated with PKH26-stained erythrocytes in normal conditions (top panels) or with 1 μM cytochalasin D (bottom panels). Left panels: plots of GFP intensity in the erythrocyte population. Cells associated with a merozoite (GFP+) are gated as EryA(green gate), and invaded cells are gated as EryIusing an algorithm recognizing merozoites associated with a tight-fitting PV (blue gate). (b) PKH26-stained erythrocytes non-invaded (top) or invaded by a merozoite surrounded by the duplication of PKH26 upon PV formation (bottom). A plot of the mean grey value of PKH26 (red) and GFP (green) signals per pixel is shown on the right of each image. The white arrows show the path of measured pixels. Scale bars, 2 μm. (c) Quantification of EryA(green) and EryI(blue) populations in the assay described inarepresented as percentages of parasites from initial input. Results are mean±s.d. from three independent experiments. (d) EryA(green) and EryI(blue) scored for WT or AMA1KOmerozoites isolated from blood cultures and incubated with erythrocytes for 10 min. Data show mean±s.d. of triplicates, representative of two independent experiments. (e) EryA(green) and EryI(blue) scored for WT or AMA1KOmerozoites isolated from blood cultures and incubated with erythrocytes for 3 min. Data show the mean of two independent experiments. KO, knockout. Figure 5: IFC analysis of erythrocyte invasion by AMA1 KO merozoites. ( a ) WT GFP + merozoites isolated from blood cultures were incubated with PKH26-stained erythrocytes in normal conditions (top panels) or with 1 μM cytochalasin D (bottom panels). Left panels: plots of GFP intensity in the erythrocyte population. Cells associated with a merozoite (GFP + ) are gated as Ery A (green gate), and invaded cells are gated as Ery I using an algorithm recognizing merozoites associated with a tight-fitting PV (blue gate). ( b ) PKH26-stained erythrocytes non-invaded (top) or invaded by a merozoite surrounded by the duplication of PKH26 upon PV formation (bottom). A plot of the mean grey value of PKH26 (red) and GFP (green) signals per pixel is shown on the right of each image. The white arrows show the path of measured pixels. Scale bars, 2 μm. ( c ) Quantification of Ery A (green) and Ery I (blue) populations in the assay described in a represented as percentages of parasites from initial input. Results are mean±s.d. from three independent experiments. ( d ) Ery A (green) and Ery I (blue) scored for WT or AMA1 KO merozoites isolated from blood cultures and incubated with erythrocytes for 10 min. Data show mean±s.d. of triplicates, representative of two independent experiments. ( e ) Ery A (green) and Ery I (blue) scored for WT or AMA1 KO merozoites isolated from blood cultures and incubated with erythrocytes for 3 min. Data show the mean of two independent experiments. KO, knockout. Full size image As additional mutations, compensatory or adverse, might accumulate in the AMA1 KO parasites propagated for extended times (up to 30 days) before IFC analysis, we next characterized AMA1 KD merozoites generated by Flippase (Flp)/Flp Recombination Target ( FRT )-mediated recombination [27] immediately before IFC ( Fig. 6a ). In this approach, AMA1 KD mosquito-stage sporozoites normally invade hepatocytes and transform into AMA1 KD hepatic merozoites [27] . The latter cannot accumulate compensatory mutations before IFC, as they are generated in the absence of selection pressure and following a single invasion/multiplication cycle. We first analysed control hepatic merozoites. IFC analysis shows that ~44.3% and ~4.1% of control GFP + hepatic merozoites score as Ery A and Ery I , respectively, indicating that erythrocytic and hepatic merozoites bind and invade erythrocytes with similar efficiency in this assay. We then used AMA1 KD hepatic merozoites, composed of ~85% of excised AMA1 − parasites lacking any detectable AMA1 and ~15% of non-excised AMA1 + individuals used as internal controls ( Fig. 6b ). IFC analysis after AMA1 immunostaining ( Fig. 7a ) shows that ~48.8% and ~5.3% of AMA1 + controls score as Ery A and Ery I , respectively, indicating that they behave like the WT ( Fig. 7b ). In contrast, only ~3.3% of AMA1 − merozoites score as Ery A ( Fig. 7b ), that is, ~15-fold less than internal controls, demonstrating a major role of AMA1 in merozoite attachment. As expected, AMA1 − merozoites also generate Ery I events after 10 min ( Figs. 6c and 7b ) or 3 min incubation ( Fig. 7c ). Remarkably, Ery I events are approximately fivefold less frequent in AMA1 − than AMA1 + merozoites when normalized to input merozoites, but approximately threefold more frequent in AMA1 − merozoites when normalized to attached parasites ( Fig. 7b , P <0.01, two-tailed t -test). Therefore, as with the Toxoplasma tachyzoite, AMA1 favours Plasmodium merozoite attachment to, but not internalization into, the host cell. 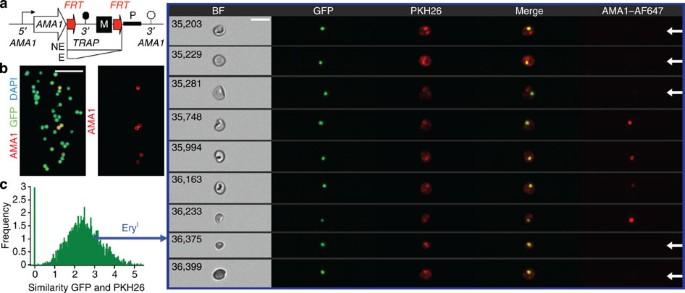Figure 6: Isolation of AMA1KDmerozoites and interaction with erythrocytes imaged by IFC. (a) Schematic illustration of theAMA1locus in Flp-expressing deleter parasites for the knockdown strategy. TwoFRTsites (red arrows) flank the 3′ UTR ofAMA1, which is excised specifically in mosquito stages when the Flp recombinase is expressed27. NE, non-excised; E, excised. (b) AMA1 immunostaining of a mixture of AMA1−(excised) and AMA1+(non-excised) merozoites isolated from HepG2 cells infected with the AMA1KDsporozoite population. Scale bar: 10 μm. (c) Hepatic merozoites frombincubated with erythrocytes and analysed by IFC. A histogram of the EryA(green) population is shown, from which the EryI(blue) is gated. Pictures of events from the EryIpopulation are shown on the right. Each line represents one acquired event. Columns from left to right: bright field (BF) and event number assigned by the IFC software; GFP (merozoite) signal; PKH26 signal; merge of GFP and PKH26 signals; AMA1 stained with Alexa-Fluor 647 (AMA1-AF647). White arrows indicate the AMA1−individuals among AMA1KDmerozoites. Scale bar, 10 μm. DAPI, 4′,6-diamidino-2-phenylindole. Figure 6: Isolation of AMA1 KD merozoites and interaction with erythrocytes imaged by IFC. ( a ) Schematic illustration of the AMA1 locus in Flp-expressing deleter parasites for the knockdown strategy. Two FRT sites (red arrows) flank the 3′ UTR of AMA1 , which is excised specifically in mosquito stages when the Flp recombinase is expressed [27] . NE, non-excised; E, excised. ( b ) AMA1 immunostaining of a mixture of AMA1 − (excised) and AMA1 + (non-excised) merozoites isolated from HepG2 cells infected with the AMA1 KD sporozoite population. Scale bar: 10 μm. ( c ) Hepatic merozoites from b incubated with erythrocytes and analysed by IFC. A histogram of the Ery A (green) population is shown, from which the Ery I (blue) is gated. Pictures of events from the Ery I population are shown on the right. Each line represents one acquired event. Columns from left to right: bright field (BF) and event number assigned by the IFC software; GFP (merozoite) signal; PKH26 signal; merge of GFP and PKH26 signals; AMA1 stained with Alexa-Fluor 647 (AMA1-AF647). White arrows indicate the AMA1 − individuals among AMA1 KD merozoites. Scale bar, 10 μm. DAPI, 4′,6-diamidino-2-phenylindole. 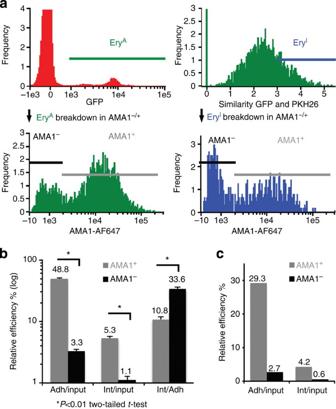Figure 7: IFC analysis and quantification of erythrocyte invasion by AMA1KDmerozoites. (a) EryAand EryIpopulations (top panels) after 10 min incubation of the AMA1KDmerozoites with PKH26-stained erythrocytes. Bottom panels show the breakdown of EryAand EryIevents in AMA1+(grey) and AMA1−(black) parasites, as measured by intensity plot of AMA1 stained with Alexa-Fluor 647 (AMA1-AF647). (b) Quantification of AMA1+(grey) and AMA1−(black) parasites in the EryAand EryIpopulations after 10 min incubation, represented as percentages of initial input parasites (Adh/Input and Int/Input, respectively), and in the EryIpopulation as percentage of adherent (EryA) parasites (Int/Adh). Results are mean±s.d. from three independent experiments. *P-value <0.01 in two-tailed Student’st-test. (c) Quantification of AMA1+(grey) and AMA1−(black) parasites in the EryAand EryIpopulations after 3 min incubation, represented as percentages of initial input parasites (Adh/Input and Int/Input, respectively). Data show the mean of two independent experiments. Full size image Figure 7: IFC analysis and quantification of erythrocyte invasion by AMA1 KD merozoites. ( a ) Ery A and Ery I populations (top panels) after 10 min incubation of the AMA1 KD merozoites with PKH26-stained erythrocytes. Bottom panels show the breakdown of Ery A and Ery I events in AMA1 + (grey) and AMA1 − (black) parasites, as measured by intensity plot of AMA1 stained with Alexa-Fluor 647 (AMA1-AF647). ( b ) Quantification of AMA1 + (grey) and AMA1 − (black) parasites in the Ery A and Ery I populations after 10 min incubation, represented as percentages of initial input parasites (Adh/Input and Int/Input, respectively), and in the Ery I population as percentage of adherent (Ery A ) parasites (Int/Adh). Results are mean±s.d. from three independent experiments. * P -value <0.01 in two-tailed Student’s t -test. ( c ) Quantification of AMA1 + (grey) and AMA1 − (black) parasites in the Ery A and Ery I populations after 3 min incubation, represented as percentages of initial input parasites (Adh/Input and Int/Input, respectively). Data show the mean of two independent experiments. Full size image AMA1 has no role in P. berghei sporozoite infection of hepatocytes Recent work using P. berghei AMA1 KD and RON4 KD sporozoites revealed strikingly distinct phenotypes, with essential and dispensable roles for RON4 and AMA1, respectively, during sporozoite invasion of hepatocytes [27] . To test AMA1 KO sporozoite capacity to invade hepatocytes, populations of GFP + AMA1 KO /GFP − AMA1 + parasites were transferred to mosquitoes. The same ratio of GFP + versus GFP − sporozoites is found in the blood fed to mosquitoes and in the mosquito salivary glands, indicating that AMA1 has no detectable effect on parasite development in the mosquitoes ( Fig. 8a ). The capacity of these salivary gland sporozoites to invade cultured hepatocytes was then tested. After sporozoite incubation with HepG2 cells in vitro , a similar proportion of AMA1 KO versus GFP − AMA1 + parasites is found in the input sporozoites and in hepatic schizonts developing inside HepG2 cells 60 h post infection ( Fig. 8b ). Likewise, in co-infection experiments of HepG2 cells with RFP + AMA1 + as control, AMA1 KO sporozoites display similar invasive capacity as the control ( Fig. 8c ). 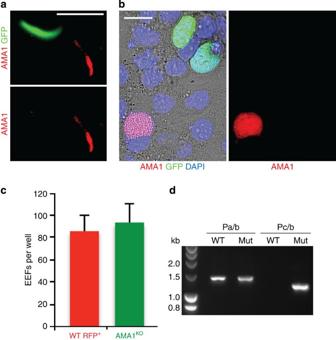Figure 8:In vitroandin vivoinfectivity of AMA1KOsporozoites. (a) AMA1 immunostaining of sporozoites dissected from mosquitoes fed with the pyrimethamine-resistant population of GFP+AMA1KO/GFP−AMA1+parasites. Scale bar, 10 μm. (b) AMA1 immunostaining of hepatic schizonts 62 h after infection of HepG2 cells by sporozoites froma. Scale bar, 20 μm. (c) Quantification of exo-erythrocytic forms (EEFs, liver stages) developing in HepG2 cells infected with GFP+(AMA1KO) or WT RFP+. Data show mean±s.d. of EEFs per well as counted in 6 wells of a 96-well plate. (d) Diagnostic PCR of the pyrimethamine-resistant population that appears in the blood of mice after intravenous injection of sporozoites froma. Pa/b pair of primers is specific for the WT locus, and Pc/b is specific for the mutant (Mut) locus. Primers are illustrated inFig. 4a. DAPI, 4′,6-diamidino-2-phenylindole. Figure 8: In vitro and in vivo infectivity of AMA1 KO sporozoites. ( a ) AMA1 immunostaining of sporozoites dissected from mosquitoes fed with the pyrimethamine-resistant population of GFP + AMA1 KO /GFP − AMA1 + parasites. Scale bar, 10 μm. ( b ) AMA1 immunostaining of hepatic schizonts 62 h after infection of HepG2 cells by sporozoites from a . Scale bar, 20 μm. ( c ) Quantification of exo-erythrocytic forms (EEFs, liver stages) developing in HepG2 cells infected with GFP + (AMA1 KO ) or WT RFP + . Data show mean±s.d. of EEFs per well as counted in 6 wells of a 96-well plate. ( d ) Diagnostic PCR of the pyrimethamine-resistant population that appears in the blood of mice after intravenous injection of sporozoites from a . Pa/b pair of primers is specific for the WT locus, and Pc/b is specific for the mutant (Mut) locus. Primers are illustrated in Fig. 4a . DAPI, 4′,6-diamidino-2-phenylindole. Full size image Finally, the infectivity of AMA1 KO sporozoites was tested in vivo . We found that intravenous injection into mice of as few as 500 AMA1 KO /AMA1 + sporozoites ( Fig. 8d ) or HepG2 cell-released hepatic merozoites (not shown) is sufficient to generate blood-stage parasite populations containing AMA1 KO parasites, demonstrating that parasites can complete a life cycle without producing AMA1. Moreover, injection into mice of only 50 AMA1 KO /AMA1 + infected erythrocytes is also sufficient to produce AMA1 KO -containing blood-stage populations (not shown). However, attempts of cloning AMA1 KO parasites were unsuccessful. This is likely due to the slower increase in parasitemia of AMA1 KO parasites, delaying the emergence of an AMA1 KO population that is eventually cleared by the mouse immune system before being detectable. Nonetheless, we cannot rule out the formal hypothesis that AMA1 KO parasites cannot be cloned because they require soluble AMA1 secreted from the AMA1 + counterparts. However, this hypothesis of AMA1 as an essential diffusible factor appears unlikely, as AMA1 KO growth is observed after co-injection of less than 50 blood stages and 500 sporozoites in the whole animal. We have inactivated AMA1 both in Toxoplasma and Plasmodium using diCre- loxP -mediated recombination and direct gene targeting, respectively, and found that AMA1-deficient T. gondii tachyzoites and P. berghei merozoites and sporozoites were still invasive and displayed a normal host cell penetration step. The most striking phenotype is that of AMA1 KO sporozoites, which showed no defect in hepatocyte invasion, confirming prior data obtained with AMA1 KD sporozoites that invaded hepatocytes even better than the WT [27] . This now demonstrates that AMA1 is dispensable for hepatocyte invasion and that, given the essential role of RON4 in the process [27] , the RON complex acts in an AMA1-independent manner. The lack of an invasion phenotype of AMA1 KO sporozoites strongly suggests that AMA1 is not involved in TJ function. In contrast to sporozoites, AMA1-deficient merozoites and tachyzoites displayed an approximately three- to fivefold decrease in overall invasion efficiency. However, like sporozoites, they penetrated host cells like the WT. They formed a normal constriction and a normal RON ring at the TJ, and tachyzoites were internalized at the normal average speed of ~20 s. Moreover, quantitative IFC analysis indicated that AMA1 KD merozoites invaded erythrocytes better than controls when normalized to adherent merozoites, reminiscent of the increased infectivity of AMA1 KD sporozoites. The decrease in invasion efficiency of AMA1-deficient tachyzoites and merozoites, which showed no defect in host cell penetration, was associated with altered zoite adhesion to host cells. Fewer AMA1-deficient merozoites bound to erythrocytes in IFC experiments, including in 3′ adhesion assays. Lack of AMA1 only modestly reduced the numbers of bound tachyzoites but affected their positioning onto cells, with AMA1-deficient tachyzoites more frequently adopting an upward position when compared with controls. AMA1 might thus be important in a pre-invasive zoite orientation step, as earlier proposed for merozoites [39] . A gradient of AMA1 on the zoite surface might create a gradient of interaction forces in a Velcro-like mechanism that might either apically reorient a zoite-expressing AMA1 mostly at its front end (merozoite) or flatten a zoite-expressing AMA1 all over its surface (tachyzoite). Why AMA1 has zoite-dependent contributions is unclear but might be related to zoite shape. A zoite-specific optimal positioning step, possibly involved in inducing rhoptry secretion, might be useful for the pear-shaped tachyzoites and merozoites and dispensable or even inhibitory for the naturally flattened sporozoites. Therefore, genetic data indicate a model where AMA1 and the RON proteins have separate roles during apicomplexan invasion. AMA1 acts in a host cell-binding step that impacts the frequency but not quality of RON-dependent TJ formation, and the AMA1–RON2 interaction is not involved in the transduction of the force generated by the zoite motor during invasion. It can be argued that our data are still compatible with an essential function of AMA1 at the TJ, if the residual invasion capacity of AMA1 mutants is ensured by an AMA1-like, functionally redundant protein. This hypothesis is highly unlikely for several reasons. First, the invasive AMA1 mutants displayed a normal entry phenotype including a fully functional TJ. This implies that any compensatory mechanism would need to be of optimal efficiency but expressed in only a subset of mutants (those that invade), a situation different from classical compensation by a suboptimal homolog that affects phenotype quality in all mutant parasites. Second, P. berghei AMA1 KD sporozoites generated by Flp/ FRT -mediated 3′-untranslated region (UTR) excision and T. gondii AMA1 KD tachyzoites generated by Tet-mediated transcriptional repression were silenced immediately before phenotype analysis, thus precluding any selection of compensatory mechanism(s). Interestingly, AMA1 KO T. gondii tachyzoites grown in continuous culture, which adapted by overexpressing the AMA1 homologue TgME49_300130 by ~15-fold ( Fig. 1d ), displayed a significantly milder adhesion phenotype, suggesting that the AMA1 homologue indeed compensated the adhesion defect of AMA1 mutants. The hypothesis of compensation at the TJ is also highly improbable in Plasmodium , which contains a single AMA1 gene. The parasite product most closely related to AMA1 is the transmembrane protein MAEBL [40] , which in P. berghei is only detected in oocyst sporozoites where it confers binding to the mosquito salivary glands but not invasion of hepatocytes [41] . Therefore, rather than AMA1-complementing TJ components, AMA1-related proteins in both Toxoplasma and Plasmodium appear to function in zoite adhesion, like AMA1. One question raised by the model in which AMA1 and the RON proteins have dissociated functions is the role of the AMA1–RON2 interaction. The interaction is not essential but is important, being evolutionarily conserved. It might be required for processing/cleavage of surface AMA1 passing the TJ, perhaps allowing the disengagement of interaction of AMA1 with its host cell receptor and facilitating zoite sliding free into the PV. Interestingly, AMA1 undergoes a conformational change upon RON2 binding [17] , which could lead to loss of adhesive function or exposure of cleavage sites. This would reconcile the genetic data and the fact that antibodies or small molecules that inhibit the interaction can reduce zoite invasion [9] , [10] , [14] , [15] , [16] , [18] , [24] , [42] . The increased frequencies of Plasmodium merozoite (relative to adhesive parasites) and sporozoite invasion might also point to a modulatory/inhibitory role, possibly in preventing other interactions important for TJ formation. More work is needed to understand the exact contribution of the AMA1–RON2 interaction, which appears to impact AMA1 but not the TJ per se . The demonstration of the dispensability of AMA1 in any step of host cell invasion by apicomplexan zoites does not question the potential efficacy of AMA1 as target of malaria prevention measures. A large body of work shows the efficacy of antibodies to AMA1 in blocking erythrocyte infection [43] , [44] , [45] , which might also reduce sporozoite invasion of hepatocytes [46] . Likewise, although the AMA1–RON2 interaction might not have any positive role in invasion, its inhibition by small molecules might still efficiently perturb invasion. Nonetheless, our finding that AMA1-less variants would be only partially impaired in adhesion while retaining normal if not increased invasive capacity, raises the possibility of rapid parasite adaptation to intervention strategies targeting only AMA1 or the AMA1–RON2 interaction. Parasites P. berghei WT ANKA strain GFP fluorescent (GFP@HSP70) [36] , RFP fluorescent (L733) [35] , AMA1/Cond [27] or AMA1 KO were maintained in 3-week-old female Wistar rats or 3-week-old female Swiss mice. Mice or rats were infected with P. berghei parasites by intraperitoneal or intravenous injections. Parasitemia was followed daily by blood smears and FACS analysis. Anopheles stephensi (Sda500 strain) mosquitoes were reared at the Centre for Production and Infection of Anopheles (CEPIA) at the Pasteur Institute as described [47] . HepG2 cell for sporozoite infection were cultured in Dulbecco’s modified Eagle’s medium (DMEM) or McCoy’s 5A medium supplemented with 10% fetal calf serum and neomycin (50 μg ml −1 , Sigma). T. gondii tachyzoites were cultured in human HFF cells maintained in DMEM supplemented with 10% fetal calf serum, 2 mM glutamine and 25 μg ml −1 gentamicin. All experiments using rodents were performed in accordance with the guidelines and regulations of the Pasteur Institute and are approved by the Ethical Committee for Animal Experimentation. Cloning of DNA constructs To generate the plasmid pGFP-hDHFR-PbAMA1 KO , the 3′UTR of Pb ama1 was amplified from P.berghei genomic DNA (gDNA) with primers 3′UTR PbAMA1 fw/rv and cloned in sites Pst I and Xho I in a modified pUC18 plasmid containing a new multiple cloning site and a human dihydrofolate reductase (hDHFR) cassette [48] (plasmid BGP-F). The 5′UTR of Pb ama1 was amplified with primers 5′UTR PbAMA1 fw/rv and cloned in sites Sac I and Eco RI in a pUC18 plasmid containing GFP@HSP70 cassette [36] in sites Sal I and Sac I. Finally, 3′UTR-hDHFR was removed from the previous plasmid and cloned in the latter in sites Pst I and Sal I. To generate p5RT70- loxP AMA1 loxP -YFP-HXGPRT, the Tg AMA1 open reading frame (ORF) was amplified from T. gondii gDNA using primers TgAMA1 ORF fw/rv. In addition, 5′UTR and 3′UTR of ama1 was amplified from T. gondii gDNA using 5′UTR TgAMA1 fw/rv or 3′UTR TgAMA1 fw/rv, respectively. First, the 5′UTR of Tg AMA1 was inserted upstream of p5RT70 in p5RT70- loxP KillerRed loxP -YFP-HXGPRT plasmid [33] in Apa I restriction sites. Then, the killerRed ORF was exchanged by Tg AMA1 ORF using Eco RI and Pac I. Finally, the 3′UTR of Tg AMA1 was cloned in after HXGPRT selection cassette using Sac I restriction sites. Transfections and selection P. berghei genetic manipulation was performed as described [49] . P. berghei AMA1 KO were generated by double homologous recombination to replace the endogenous ama1 -coding sequence by a hDHFR cassette [48] and a GFP fluorescence cassette [36] . The targeting sequence with the two homologous regions flanking the selection cassettes was PCR amplified from plasmid pGFP-hDHFR-PbAMA1 KO using primers 5′UTR PbAMA1 fw and 3′UTR PbAMA1 rv, and gel purified using the NucleoSpin Gel and PCR Clean-up kit (Macherey-Nagel) following kit instructions. After transfection of an enriched preparation of P. berghei ANKA schizonts and re-injection into mice, mutants were selected with constant treatment with pyrimethamine in drinking water until green fluorescent parasitemia was detected. Drugs were used as described [49] . The presence of AMA1 KO was confirmed by PCR analysis with primers Pa/Pb, specific for the WT ama1 locus, and Pb/Pc, specific for integration at the ama1 locus, and by Southern blotting of total gDNA after digestion with the restriction enzymes Mfe I or Nde I, with a probe hybridizing at the 5′UTR of ama1 , amplified with primers 5′Pb ama1 -probe fw/rv, to recognize the WT or the mutant loci with different sizes. For T. gondii genetic manipulation, ca 1 × 10 7 of freshly lysed parasites were transfected with 60 μg linearized DNA by electroporation. Selection was performed with mycophenolic acid (12.5 mg ml −1 in MeOH) and xanthine (20 mg ml −1 in 1 M KOH) [50] , or phleomycin (50 μg ml −1 ) [51] . The TgAMA1 IoxP strain was generated by replacement of the endogenous ama1 by floxed ama1 via homologous recombination. The targeting sequence p5RT70- loxP AMA1 loxP -YFP-HXGPRT was removed from plasmid by digestion with Nsi I and Xma I restriction enzymes and transfected into ku80::diCre recipient strain [33] . Parasites with stable integration were selected by the treatment with xanthine and mycophenolic acid. Integration by homologous recombination was confirmed by 5′TgAMA1out fw (P1) and p5RT70 rv (P1′) primers. In addition, a PCR with TgAMA1int fw (P2) and TgAMA1 ORF rv (P2′) primers was conducted to discriminate the presence of genomic or coding sequence of ama1 ORF. To generate TgAMA1 KO , amal ORF was excised from the genome by activation of diCre with 50 nM rapamycin for 16 h. Subsequent limited dilution of induced TgAMA1 loxP pool led to a clonal TgAMA1 KO population, which was confirmed by genomic PCR using primers upstream and downstream of the loxP sites, 5′UTR TgAMA1 fw (P3) and YFP rv (P3′). The loss of ama1 ORF was further verified by a PCR in the ORF with primers TgAMA1int fw (P2) and TgAMA1 ORF rv (P2′). For complementation studies, TgAMA1 FLAG [52] was used. Southern and western blotting gDNA from P. berghei and T. gondii to use as a PCR template and for Southern blotting was extracted using Qiagen dneasy blood and tissue kit according to manufacturer’s protocol. For Southern blotting of P. berghei gDNA, samples were digested with Mfe I or Nde I restriction enzymes overnight, precipitated with ethanol, washed and separated in agarose gel. The gel was transferred to a Hybond-XL membrane (GE-Healthcare) and blotting was performed using the DIG easy Hyb kit and DIG wash and block buffer kit from Roche according to manufacturer’s protocol. The probe was amplified with primers 5′Pb ama1 -probe fw/rv using the DIG Probe Synthesis kit from Roche. Tachyzoite western blot samples were obtained by spinning down extracellular parasites and incubating with RIPA buffer (50 mM Tris-HCl pH 8; 150 mM NaCl; 1% Triton X-100; 0.5% sodium deoxycholate; 0.1% SDS; 1 mM EDTA) for 20 min on ice. Unless indicated otherwise 10 6 parasites were loaded onto a SDS acrylamide gel and immunoblot was performed as previously described [53] . Briefly, proteins were transferred onto a nitrocellulose membrane, after blocking the membranes were incubated with primary antibody for 1 h (mouse anti-AMA1 1:1,000; rabbit anti-aldolase 1:10,000) followed by incubation with horseradish peroxidase-labelled secondary antibodies (1:50,000; Jackson ImmunoResearch) for 2 h. Table 1 Primers used in this study. Full size table Quantitative PCR RNA from freshly egressed parasites was purified using Trizol followed by chloroform extraction. For cDNA synthesis, 2.5 μg of total RNA were retrotranscribed using the SuperScript VILO (Invitrogen, Life Technology). Quantitative real-time PCR was performed on a LightCycler 480 (Roche) using the LightCycler 480 SYBR Green I Master Mix (Roche). PCR primers were designed to amplify a 100-bp target gene fragment: AMA1 Fw: 5′-TGGAGAGAACCCAGATGCGTTCCT-3′; AMA1 Rv: 5′-CAGTGTAGTCGAGGCAACGGCC-3′; TgME49_300130 Fw: 5′-CCAGGACACGATGCCGCTCG-3′; TgME49_300130 Rv: 5′-AACCCCTCCGCCTCGTCCTT-3′. cDNA levels were normalized to α-tubulin levels measured with primers: Fw: 5′-GCATGATCAGCAACAGCACT-3′; Rv: 5′-ACATACCAGTGGACGAAGGC-3′. Experiments were performed four times with two different RNA preparations. Immunofluorescence For P. berghei merozoites, sporozoites and infected HepG2 cells immunofluorescence, samples were fixed with 4% paraformaldehyde, 0.0075% glutaraldehyde in PBS for 1 h [54] , permeabilized with 0.1% Triton X-100 in PBS, blocked with BSA 3% in PBS, and stained with primary rabbit polyclonal antibodies to the P. berghei AMA1 peptide CRASHTTPVLMQKPYY (Eurogentec, 1:500 dilution), or primary polyclonal antibodies to the P. berghei RON2 peptide KKLGKLREKIVNGLFKKRGK (Thermo Scientific, 1:500 dilution), followed by secondary Alexa-Fluor-conjugated antibodies (Molecular Probes, 1:500 dilution). Images were acquired using an Axiovert II fluorescence microscope (Zeiss) or the ImageStreamX from AMNIS. For T. gondii immunofluorescence analysis, infected HFF monolayers grown on coverslips were fixed in 4% paraformaldehyde for 20 min at room temperature, followed by permeabilization (0.2% Triton X-100 in PBS) and blocking (2% BSA and 0.2% Triton X-100 in PBS). The staining was performed using primary antibody (mouse anti-AMA1, 1:1,000; mouse anti-SAG1, 1:1,000; rabbit anti-MIC2, 1:500; rabbit anti-IMC1, 1:1,500; rabbit anti-GAP45 1:1,000) followed by secondary Alexa-Fluor-conjugated antibodies (Molecular Probes, 1:3,000). Images were acquired with CCD camera under Deltavision Core or confocal Nikon Ti eclipse microscopes (z–stacks of 0.2–0.3 μm, × 100 immersion objective), deconvolved using SoftWoRx Suite 2.0 (Applied Precision, GE) when needed and further processed using ImageJ 1.34r and Photoshop (Adobe Systems) software. Production of merozoites and ImageStream analysis Erythrocytic merozoites were obtained by culturing infected rat or mouse blood for 16 h, at 37 °C, 5% CO 2 and 10% O 2 , under shaking (90 r.p.m. ), in RPMI 1,640 medium (Gibco) supplemented with 20% fetal calf serum and 50 μg ml −1 neomycin. Mature schizonts were separated in a Nycodenz gradient and merozoites were isolated by filtration of schizonts through a 5-μm filter, followed by another filtration through a 1.2-μm filter. The GFP fluorescent AMA1 KD strain conditionally knocks down AMA1 expression in mosquito stages, producing sporozoite populations in mosquito salivary glands in which up to 95% of the parasites express undetectable levels of AMA1 (ref. 27 ). AMA1 KD sporozoites were used to infect HepG2 cell in vitro and 62 h post infection the emerging merosomes were collected, and hepatic merozoites were obtained by filtration through a 5-μm filter. The purified merozoites were cultured in vitro with PKH26-stained rat red blood cells for 3 or 10 min under agitation (400 r.p.m. ), and cultures were fixed with 4% paraformaldehyde, 0.0075% glutaraldehyde in PBS for further permeabilization and staining with anti-AMA1 (Eurogentec, peptide CRASHTTPVLMQKPYY) and secondary Alexa-Fluor 647. Cells were acquired in an ImageStream X using a × 60 objective, excitation lasers 488, 561 and 642 nm, and analysed using the software IDEAS, from AMNIS. Merozoites attached to red blood cells were assessed by double fluorescence (PKH26 and GFP), and invaded cells were assessed with a sequence of algorithms that identify PKH26 duplication because of PV formation (R3 Bright Similarity Channels 2 and 4, Intensity Weighted). T. gondii invasion/attachment assay To investigate the attachment and invasion rates of the TgAMA1 KO parasites, a red/green invasion assay was performed as described earlier [55] . HFFs were grown on coverslips of a 24-well plate and infected with 5 × 10 6 freshly collected parasites. Plates were centrifuged for 2 min at 200 g and incubated at 37 °C, 5% CO 2 for 15 min. Subsequently, cells were fixed in 4% paraformaldehyde (PFA) for 15 min followed by immunostaining with α-SAG-1 primary and Alexa-Fluor secondary antibodies before Triton X-100 permeabilization (0.2% in PBS) and immunostaining with α-IMC1 primary and Alexa-Fluor secondary antibodies. Extracellular and intracellular parasites were counted in ten fields of view (× 100 objectives) and calculated as a percentage value of RH Δhxgprt parasites normalized to 100%. To measure T. gondii tachyzoite position relative to the host cell, we adapted the assay previously described [27] . HeLa cells were plated on poly-lysine-coated glass coverslips in a 6-well plate, transfected with 1 μg of plasmid-encoding mCherry in the pDisplay Vector (Invitrogen) and used 20 h later for a 5-min invasion assay. Cells were fixed in PBS-4% PFA (20 min, room temperature) and stained with anti-SAG-1 antibodies followed by Alexa-Fluor anti-mouse antibodies to label extracellular parasites. Samples were scanned on the confocal Nikon Ti Eclipse microscope and images were captured and analysed with Metamorph software (using the 4D viewer application). For each zoite, an ellipsoid was fit to measure the longitudinal axis, whereas the cell surface contacting the tachyzoite centres of mass was affected to all the isosurfaces. The plane of the cell was reconstructed and angle values between the longer axis of the parasite and the host cell plane were generated by Metamorph. T. gondii replication assay 1 × 10 5 ku80::diCre or TgAMA1 FLAG or 5 × 10 5 TgAMA1 KO were inoculated onto a confluent monolayer of HFFs grown on coverslips (24-well plate) and incubated in normal growth conditions. One hour post inoculation, coverslips were washed in PBS to remove extracellular parasites and thus synchronize the cell cycle. Cells were further grown in normal growth conditions until as indicated, fixed and immunostained. The number of parasites per vacuole was determined for 100 vacuoles. T. gondii plaque assay 200 RH Δhxgprt or TgAMA1 FLAG parasites or 1,000 TgAMA1 KO parasites were added onto a confluent monolayer of HFF cells of a six-well plate. After incubating for 6 days, the HFF monolayer was washed in PBS and fixed in ice-cold methanol for 20 min. Afterwards, the HFF cells were stained with Giemsa. The area of ten plaques was assessed using Image J 1.34r software. T. gondii egress assay 4 × 10 5 parasites were grown in HFF monolayers on coverslips for 36 h. Media were exchanged for pre-warmed, serum-free DMEM supplemented with calcium ionophore 2 μM (A23187 in DMSO) [56] . After incubation for 5 min at normal growth conditions (37 °C; 5% CO 2 ), cells were fixed and stained with anti-GAP45 primary antibody and Alexa-Fluor secondary antibody. Two hundred vacuoles were scored in each experiment. T. gondii motility assay Freshly egressed tachyzoites were allowed to glide for 30 min on glass coverslips coated with 50 μg ml −1 heparin in PBS. Parasites and trails were then stained with anti-P30 antibodies and visualized with an inverted laser scanning microscope (Eclipse Ti, Nikon). Images were analysed using Metamorph and ImageJ software. Numbers of helical and circular trails associated with parasites were scored in 30 fields. T. gondii video microscopy Time-lapse video microscopy was conducted with the DeltaVision® Core microscope using a × 40 immersion lens. Freshly lysed RH Δhxgprt, ku80::diCre or TgAMA1 KO were added onto HFF, HeLa or U373 monolayer grown in glass dishes (ibidi; μ-Dish 35 mm, high ). Forty hours post inoculation, invasion of freshly egressed parasites was observed. Normal growth conditions were maintained throughout the experiment (37 °C; 5% CO 2 ). Images were recorded at one frame per second. Further image processing was performed using ImageJ 1.34r software and with Photoshop (Adobe Systems). How to cite this article: Bargieri, D. Y. et al . Apical membrane antigen 1 mediates apicomplexan parasite attachment but is dispensable for host cell invasion. Nat. Commun. 4:2552 doi: 10.1038/ncomms3552 (2013).